An unconventional bilayer ice structure on a NaCl(001) film Water–solid interactions are of broad importance both in nature and technology. The hexagonal bilayer model based on the Bernal–Fowler–Pauling ice rules has been widely adopted to describe water structuring at interfaces. Using a cryogenic scanning tunnelling microscope, here we report a new type of two-dimensional ice-like bilayer structure built from cyclic water tetramers on an insulating NaCl(001) film, which is completely beyond this conventional bilayer picture. A novel bridging mechanism allows the interconnection of water tetramers to form chains, flakes and eventually a two-dimensional extended ice bilayer containing a regular array of Bjerrum D-type defects. Ab initio density functional theory calculations substantiate this bridging growth mode and reveal a striking proton-disordered ice structure. The formation of the periodic Bjerrum defects with unusually high density may have a crucial role as H donor sites in directing multilayer ice growth and in catalysing heterogeneous chemical reactions on water-coated salt surfaces. The interactions of water with the surfaces of solid materials are crucial for a great many environmental, biophysical and even technological processes [1] . Conventionally, the hexagonal bilayer model based on the Bernal–Fowler–Pauling ice rules has been widely adopted to describe water structuring at various interfaces [2] . This hexagonal ice-like bilayer consists of a puckered hexagonal overlayer with water molecules located at two distinct heights, where the lower water molecules donate two hydrogen bonds (H bonds) to the upper layer and bond relatively strongly with the substrate, whereas the higher-lying molecules provide one donor H bond to the bottom layer and do not interact appreciably with the substrate. Recent molecular-level studies on water/metal interfaces reveal that water is distorted from the conventional bilayer-like arrangement and exhibits remarkably rich H-bonded structures arising from a subtle balance between the water–water and water–metal interactions [2] , [3] , [4] , [5] , [6] , [7] , [8] , [9] , [10] , [11] , [12] , [13] . Therefore, the validity of the hexagonal bilayer model on interfacial water is being challenged [13] . In spite of these exciting findings for water–metal interfaces, the detailed molecular-level understanding of water on insulating surfaces is still in its infancy. Water structuring on the insulating surfaces is more intriguing but more challenging than that on metal surfaces because of the complicated nature of water–insulator interaction [10] , [14] , [15] , [16] , [17] . Salt is one of the most widespread insulating materials in our daily life and also one of the most abundant components of atmospheric particles. Understanding water–salt interaction is of fundamental importance to many applied fields ranging from atmospheric chemistry to biology [1] , [14] , [18] , [19] . During past decades, wetting layer structures of water on salt surfaces have been studied using spectroscopic and diffraction techniques as well as ab initio theoretical calculations [20] , [21] , [22] , [23] , [24] , [25] , [26] , [27] , [28] , but the obtained information is still controversial and far from complete mainly because of the lack of ability to experimentally access the molecular-level details of water/salt interfaces. Using a cryogenic scanning tunnelling microscope (STM), here we report the molecular-level imaging of ice nucleation and growth on an Au-supported NaCl(001) film. The STM topographic images with unprecedented resolution allow us to identify a new type of two-dimensional (2D) ice-like bilayer structure built from cyclic water tetramers, which is completely beyond the conventional hexagonal bilayer model. The water tetramers within the lower part of the bilayer act as the basic building blocks on the NaCl(001) surface, which are interconnected via a novel bridging mechanism to form a regular array of Bjerrum D-type defects located in the upper layer [29] . Ab initio theoretical calculations based on density functional theory (DFT) substantiate this bridging growth mode and reveal a striking proton-disordered ice structure. The formation of the periodic Bjerrum defects with unusually high density is strongly against the Bernal–Fowler–Pauling ice rules and may have a crucial role as H donor sites in directing multilayer ice growth and in catalysing heterogeneous chemical reactions on water-coated salt surfaces. Growth of water nanoclusters on NaCl(001) islands The deposition of NaCl on a Au(111) surface at room temperature leads to the formation of bilayer (001)-terminated islands with perfect non-polar step edges via a carpet-like growth mode ( Fig. 1a ; for experimental details see Methods section) [30] , [31] . The bilayer NaCl island has a thickness of ~5.5 Å such that the electrons from STM tip are still able to tunnel through the insulating films and drain into the Au substrate. 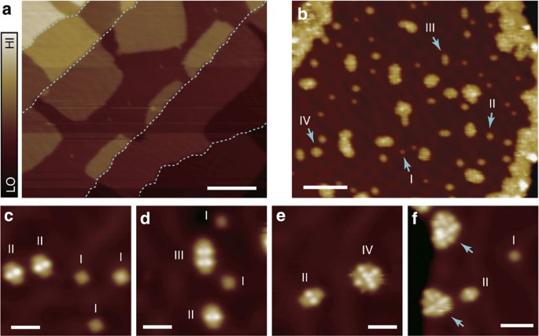Figure 1: Growth of water nanoclusters on NaCl(001) islands. (a) STM topography of bilayer NaCl(001) islands grown on the Au(111) surface acquired at 77 K. The step edges of the Au(111) surface are highlighted by the sky-blue dotted lines. Scale bar, 15 nm. (b) STM topography of a NaCl(001) island after dosing ~0.1 bilayer water molecules at 77 K. The water clusters appear in four characteristic representations (denoted as I, II, III and IV by the sky-blue arrows). Set point:V=500 mV andI=10 pA. Scale bar, 8 nm. (c–f) Zoom-in STM images of the isolated water clusters I, II, III and IV. The larger water clusters with irregular shapes are denoted by the sky-blue arrows inf. (c,e) were acquired at 77 K. (d,f) were acquired at 5 K. Set points ofc:V=20 mV andI=10 pA;d:V=100 mV andI=10 pA;e:V=20 mV andI=150 pA;f:V=100 mV andI=10 pA. Scale bars, 2 nm (c–e); 3 nm (f). HI, high; LO, low. Figure 1b shows a typical STM image focusing on a NaCl island after dosing ~0.1 bilayer water molecules at 77 K. Owing to the high mobility of water on the NaCl(001) surface, most of the water molecules aggregate at the edge of the NaCl island while isolated water clusters can form on the terrace occasionally. We note that the aggregated water clusters at the island edge can be extracted onto the terrace by injecting hot electrons into the bare Au surface near the NaCl island. Figure 1: Growth of water nanoclusters on NaCl(001) islands. ( a ) STM topography of bilayer NaCl(001) islands grown on the Au(111) surface acquired at 77 K. The step edges of the Au(111) surface are highlighted by the sky-blue dotted lines. Scale bar, 15 nm. ( b ) STM topography of a NaCl(001) island after dosing ~0.1 bilayer water molecules at 77 K. The water clusters appear in four characteristic representations (denoted as I, II, III and IV by the sky-blue arrows). Set point: V =500 mV and I =10 pA. Scale bar, 8 nm. ( c – f ) Zoom-in STM images of the isolated water clusters I, II, III and IV. The larger water clusters with irregular shapes are denoted by the sky-blue arrows in f . ( c , e ) were acquired at 77 K. ( d , f ) were acquired at 5 K. Set points of c : V =20 mV and I =10 pA; d : V =100 mV and I =10 pA; e : V =20 mV and I =150 pA; f : V =100 mV and I =10 pA. Scale bars, 2 nm ( c – e ); 3 nm ( f ). HI, high; LO, low. Full size image Most of the water clusters appear as four characteristic representations (denoted as I, II, III and IV in Fig. 1b ). Figure 1c–f presents zoom-in STM images of those isolated water clusters on the NaCl islands. These four types of clusters are regular in shape and can be recurrently found on the surface. Apparently, type-I cluster has C4 symmetry, whereas type-II, -III and -IV clusters exhibit C2 symmetry. Type-II and -III water clusters show two equivalent orientations aligning with the underlying NaCl(001) lattice. In addition, we also find larger water clusters with irregular shapes, two of which are denoted in Fig. 1f by arrows. The irregular-shaped water clusters are actually not amorphous but result from the agglomeration or coalescence of the four types of smaller clusters (see the next section). Imaging and models of the water nanoclusters High-resolution STM images of the four types of water clusters are shown in the left column of Fig. 2 . Type-I water cluster consists of four equivalent lobes, suggesting that it actually corresponds to a water tetramer lying flat on the surface ( Fig. 2a–c ). The STM images of type-II, -III and -IV water clusters exhibit interesting bilayer structures ( Fig. 2d–l ). It is evident that the lower layers of the type-II, -III and -IV water clusters are composed of two, three and four tetramers, respectively. The water molecules within the upper layers, which appear as individual protrusions, locate exactly between the corners of the neighbouring tetramers. Therefore, the planar water tetramers seem to be the basic building blocks on the NaCl(001) surface, which could be interconnected via bridging water molecules to form larger clusters. 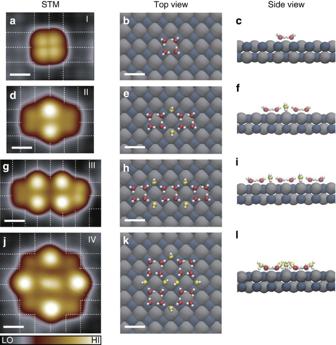Figure 2: Imaging and models of four types of water clusters. (a–c) Type-I; (d–f) type-II; (g–i) type-III; and (j–l) type-IV. (a,d,g,j) STM topographies of the water nanoclusters acquired at 5 K. Square lattices of the NaCl(001) surface arising from Cl−are depicted by white grids. Set points ofa:V=20 mV andI=50 pA;d:V=7 mV andI=550 pA;g:V=6 mV andI=400 pA;j:V=5 mV andI=120 pA. (b,e,h,k) and (c,f,i,l): Top and side views, respectively, of the calculated adsorption configurations of the water clusters. H, Cl−and Na+are denoted by white, grey and dark-cyan spheres, respectively. For clarity, the O atoms of water molecules in lower and upper layers are represented by red and yellow spheres, respectively. Scale bars 5 Å. The calculated OH-bond lengths and HOH angles are listed inSupplementary Table 2. HI, high; LO, low. Figure 2: Imaging and models of four types of water clusters. ( a – c ) Type-I; ( d – f ) type-II; ( g – i ) type-III; and ( j – l ) type-IV. ( a , d , g , j ) STM topographies of the water nanoclusters acquired at 5 K. Square lattices of the NaCl(001) surface arising from Cl − are depicted by white grids. Set points of a : V =20 mV and I =50 pA; d : V =7 mV and I =550 pA; g : V =6 mV and I =400 pA; j : V =5 mV and I =120 pA. ( b , e , h , k ) and ( c , f , i , l ): Top and side views, respectively, of the calculated adsorption configurations of the water clusters. H, Cl − and Na + are denoted by white, grey and dark-cyan spheres, respectively. For clarity, the O atoms of water molecules in lower and upper layers are represented by red and yellow spheres, respectively. Scale bars 5 Å. The calculated OH-bond lengths and HOH angles are listed in Supplementary Table 2 . HI, high; LO, low. Full size image To confirm this bridging mechanism, we carry out systematic ab initio DFT calculations (for details see Methods section) based on the STM images of the water clusters where the underlying NaCl(001) lattice is simultaneously resolved ( Fig. 2a,d,g and j ). The water molecules are adsorbed on the Na + through electric interaction ( Supplementary Note 1 and Supplementary Fig. 1 ). The tetramers observed in this work have exactly the same structure as the ones built by tip manipulation at 5 K. Our previous STM and DFT studies reveal that each water molecule donates and accepts just one H bond resulting in a cyclic tetramer, whereas the other four free OH bonds point obliquely upward away from the surface ( Fig. 2b,c ) [30] . Such a tetramer structure is similar to the one proposed in ref. 24 . It is worthy to note that the tetramer actually contains two degenerate chiral H-bonded loops, which can be distinguished through orbital imaging [30] . For the type-II cluster, the calculations reveal that two tetramers are bridged by two water molecules and each bridging molecule accepts two H bonds from the two tetramers ( Fig. 2e ). Owing to the tetrahedral-coordination structure of the water molecule, both of the two OH bonds of the bridging water molecule point outward along the short axis of the type-II cluster. One of the OH bonds points obliquely upward and the other forms H bond with the Cl − anion in the substrate ( Supplementary Note 1 ), such that the bridging water molecules are ~0.85 Å higher than the tetramers ( Fig. 2f ). This explains the larger apparent height of the bridging water molecules measured by STM. Similar effect of the orientation of water molecules on the apparent height has been observed in previous studies [8] , [9] . This bridging mechanism also allows the formation of the triple tetramer (type-III cluster) as shown in Fig. 2g–i . The type-IV water cluster consists of four tetramers interconnected via six bridging water molecules with four at the edges and two in the centre ( Fig. 2k ). Interestingly, the two inner bridging water molecules always pair up but avoid facing each other because of the repulsive force between the H atoms, forming a Bjerrum D-type defect (a crystallographic defect specific to ice, where there are two protons between the nearest-neighbour pair of oxygen atoms) [12] , [29] . The Bjerrum D-type defect has two orthogonal orientations, which can be switched reversibly by the STM tip ( Supplementary Note 2 and Supplementary Fig. 2 ). Each inner bridging water molecule donates one H bond to the Cl − in the substrate so that the Cl − is lifted up ~0.5 Å from the surface ( Fig. 2l ). The lifting of the Cl − via the H + –Cl − interaction suggests that the Cl − tends to depart before the Na + at the early stage of the salt dissolution, which is consistent with the earlier theoretical predictions [32] , [33] , [34] . We also notice that the two bridging water molecules in the centre have a lower apparent height than the four molecules at the periphery, which might arise from the stronger interaction between the two water molecules in the centre and the NaCl surface because of the lifting of the Cl − . As the water coverage further increases, larger water clusters or ice flakes can be built up via the similar bridging mechanism ( Fig. 3 ). 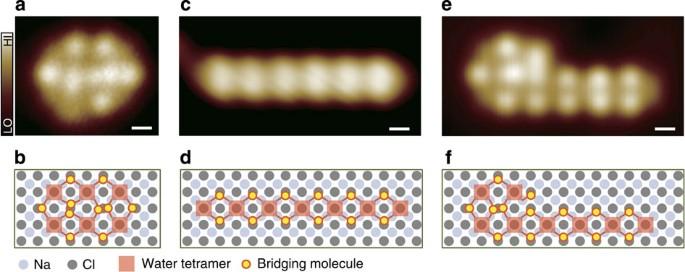Figure 3: Imaging and models of larger water clusters. (a) STM image (77 K) of a 6-tetramer ice flake. (c) STM image (77 K) of a 7-tetramer chain. (e) STM image (5 K) of a composite water cluster with an irregular shape that consists of a type-IV cluster and a 4-tetramer chain. Scale bars, 5 Å (a,c,e). (b,d,f) The schematic adsorption models corresponding to (a,c,e), respectively. The red solid squares denote the water tetramers and the yellow spheres denote the bridging water molecules. Cl−and Na+are denoted by the grey and light grey spheres, respectively. Set points ofa:V=20 mV andI=8 pA;cV=400 mV andI=8 pA;e:V=100 mV andI=20 pA. HI, high; LO, low. Figure 3a,c shows a 6-tetramer ice flake containing two Bjerrum defects and a 7-tetramer chain, respectively. The corresponding adsorption structures are schematically depicted in Fig. 3b,d . It is evident that the bridging mechanism allows both the 1D and 2D growth of the extended tetramer-based ice structures on the NaCl(001) surface. Figure 3e,f displays a more complicated ice flake with an irregular shape, which actually consists of a type-IV cluster and a 4-tetramer chain. More generally, any irregular-shaped water clusters could be identified as a certain tetramer array interconnected by bridging water molecules. Figure 3: Imaging and models of larger water clusters. ( a ) STM image (77 K) of a 6-tetramer ice flake. ( c ) STM image (77 K) of a 7-tetramer chain. ( e ) STM image (5 K) of a composite water cluster with an irregular shape that consists of a type-IV cluster and a 4-tetramer chain. Scale bars, 5 Å ( a , c , e ). ( b , d , f ) The schematic adsorption models corresponding to ( a , c , e ), respectively. The red solid squares denote the water tetramers and the yellow spheres denote the bridging water molecules. Cl − and Na + are denoted by the grey and light grey spheres, respectively. Set points of a : V =20 mV and I =8 pA; c V =400 mV and I =8 pA; e : V =100 mV and I =20 pA. HI, high; LO, low. Full size image Growth mechanism of the water nanoclusters The growth mechanism of the tetramer-based water clusters can be energetically rationalized by adsorption energy calculations using DFT. We first address the stability of the water tetramer. The adsorption energy per water molecule gradually increases from the monomer to the tetramer ( Fig. 4 ). The adsorption energies of the monomer, dimer and trimer are at least ~100 meV per H 2 O molecule smaller than that of the tetramer. From the trends of water–water and water–substrate interactions ( Fig. 4 ), one can see that the gain of the adsorption energy is mainly contributed by the increase of the water–water interaction from the monomer to the tetramer owing to the increased number of H bonds per water molecule. Other flat clusters such as pentamers or hexamers are not favoured because the number of H bonds per water molecule does not increase while the water–substrate interaction would be significantly weakened because of the symmetry mismatch. Therefore, the tetramers are the most stable clusters and correspond to the basic building blocks on the NaCl(001) surface. 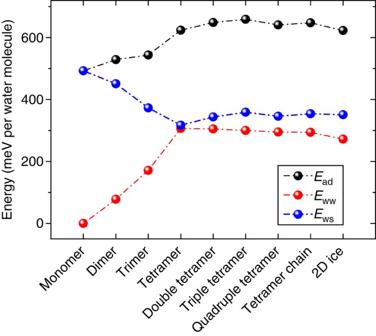Figure 4: Adsorption energy of different water clusters. Ead(black) is the total adsorption energy;Eww(red) is the water–water interaction; andEws(blue) is the water–substrate interaction (for definitions please refer to Methods section). Figure 4: Adsorption energy of different water clusters. E ad (black) is the total adsorption energy; E ww (red) is the water–water interaction; and E ws (blue) is the water–substrate interaction (for definitions please refer to Methods section). Full size image To explore the reason why the water tetramers are linked together via the bridging mechanism, we calculate the adsorption energies of double (type-II), triple (type-III), quadruple tetramer (type-IV), tetramer chain and tetramer-based 2D ice (see the next section), which are then compared with that of the isolated tetramer ( Fig. 4 ). It is clear that the adsorption energy per water molecule almost levels off from the isolated tetramer to tetramer-based larger clusters. Therefore, interconnecting the tetramers via bridging water molecules does not sacrifice the adsorption energy and is thermodynamically favourable. It is worthy to note that the bridging water molecule form H bonds with both the neighbouring water molecules and the Cl − atom in the substrate, such that both the water–water and water–substrate interactions are maximized. To gain more insight into the growth mechanism, we perform statistic analysis out of 150 different water clusters, which shows that the proportions of type-I, type-II, type-III, type-IV and those with irregular shape are 34.6%, 24.6%, 6.2%, 8.6% and 26%, respectively. It is obvious that the occurrence of the water clusters is not only governed by adsorption energies but more importantly by the size and the microscopic structure of the cluster. Therefore, the growth of the water clusters is actually kinetically limited. 2D tetragonal bilayer-like ice Further increasing the coverage, the water can eventually wet the NaCl(001) surface via such bridging mechanism. 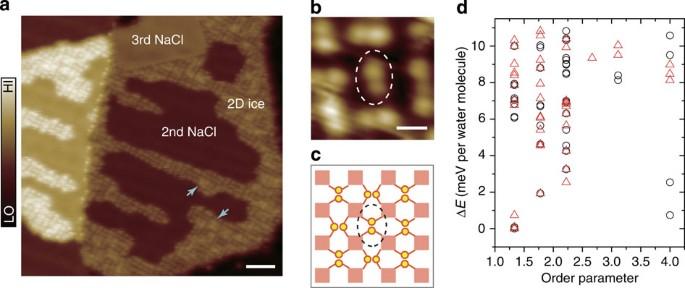Figure 5: 2D tetragonal bilayer ice on the NaCl(001) surface. (a) STM image (77 K) of the 2D ice growth on a NaCl island. The arrows denote the ice nucleation on top of the 2D ice island. Set point:V=400 mV andI=10 pA. Scale bar, 4 nm. (b) Zoom-in STM image (77 K) of the 2D ice structure. Set point:V=350 mV andI=10 pA. Scale bar, 5 Å. (c) Schematic model of the 2D tetragonal bilayer ice, corresponding tob. The red solid squares denote the water tetramers and the yellow spheres denote the bridging water molecules. The dashed white and black ellipses inbandchighlight one of the Bjerrum D-type defects. (d) Total energy difference per water molecule between different 2D ice structures as functions of two kinds of order parameter (tetramer chirality: black circle; the orientation of the Bjerrum defect: red triangle). The energy difference is with respect to the most stable adsorption structure, whose adsorption energy is 623 meV per H2O molecule. The order parameter is defined as the average number of the nearest neighbours with the same states as the one being counted. An order of 4 represents a ferro state, whereas 0 represents an anti-ferro state. HI, high; LO, low. Figure 5a shows the 2D growth of the extended water monolayer at a coverage of ~0.3 bilayer. These 2D water islands develop along the edge as well as on the terrace of the NaCl island, modulated by the herringbone reconstructions of the Au(111) surface. The zoom-in STM images ( Fig. 5b ) show that the 2D water island consists of paired protrusions, one of which is highlighted by a dashed white ellipse. Such 2D water overlayer can be considered as a tetragonal bilayer-like ice: the tetramer arrays within the lower layer are interconnected by paired bridging water molecules within the upper layer (highlighted by a dashed black ellipse in Fig. 5c ), leading to a regular array of Bjerrum D-type defects. The paired protrusions observed in Fig. 5b thus result from the Bjerrum defects within the upper layer. The tetramer arrays are not visible since they form uniform background in the STM images. Similar to the type-IV cluster, the Bjerrum defect of the 2D ice can have two orthogonal orientations but show no noticeable long-range ordering. The Bjerrum D-type defects with such high density provide an effective source of uncoordinated OH groups, which act as the active sites for the second-layer ice nucleation. Figure 5: 2D tetragonal bilayer ice on the NaCl(001) surface. ( a ) STM image (77 K) of the 2D ice growth on a NaCl island. The arrows denote the ice nucleation on top of the 2D ice island. Set point: V =400 mV and I =10 pA. Scale bar, 4 nm. ( b ) Zoom-in STM image (77 K) of the 2D ice structure. Set point: V =350 mV and I =10 pA. Scale bar, 5 Å. ( c ) Schematic model of the 2D tetragonal bilayer ice, corresponding to b . The red solid squares denote the water tetramers and the yellow spheres denote the bridging water molecules. The dashed white and black ellipses in b and c highlight one of the Bjerrum D-type defects. ( d ) Total energy difference per water molecule between different 2D ice structures as functions of two kinds of order parameter (tetramer chirality: black circle; the orientation of the Bjerrum defect: red triangle). The energy difference is with respect to the most stable adsorption structure, whose adsorption energy is 623 meV per H 2 O molecule. The order parameter is defined as the average number of the nearest neighbours with the same states as the one being counted. An order of 4 represents a ferro state, whereas 0 represents an anti-ferro state. HI, high; LO, low. Full size image The H bond chirality of the tetramer and the orientation of the Bjerrum defect could be two parameters reflecting the proton ordering in ice structures, which is of great importance to ice growth, surface corrosion, catalysis and so on [10] , [35] , [36] , [37] . To clarify this issue, we plot the relative total energy of a 2D bilayer ice as functions of the two order parameters. Taking the chirality of the tetramer as an example, this order parameter is defined as the average number of nearest-neighbour tetramers, which have the same chirality as the one being counted. In a perfectly ordered case, this value should be 4. The same definition is applied to the orientation of the Bjerrum defect. The results are shown in Fig. 5d . It is clear that the total energy differences between different ice structures fall within ~10 meV and show no dependence on either of these two order parameters. Although the water tetramers form an ordered tetragonal array in the 2D ice bilayer, the distribution of protons is actually disordered. The disordered proton distribution in the 2D ice bilayer suggests that the growth of the second layer of ice should be quite different from that on the conventional ice surface where the proton ordering has an important role [36] , [37] . STM studies reveal that water tends to form ice clusters around the Bjerrum defects on top of the 2D ice before the completion of the 2D ice bilayer (see the arrows in Fig. 5a ). Such ice clusters are disordered and never agglomerate to form ordered ice overlayer even at high water coverage. As a step towards relating the current work to realistic environmental systems, we perform systematic temperature-dependent STM studies. The 2D ice bilayer remains stable up to 145 K. Further increasing the temperature leads to dissolution and even decomposition of the bilayer NaCl islands ( Supplementary Note 3 and Supplementary Fig. 3 ). Such a behaviour might be related to the periodic Bjerrum D-type defects of the 2D ice, which lift up the Cl − ~0.5 Å from the surface via the H + –Cl − interaction ( Fig. 2l ). These results provide unprecedented opportunity for understanding the initial stage of NaCl dissolution at higher temperature, which is an important process during the formation of the water-coated NaCl aerosols. Considering that the structure of adsorbed water may depend on the amount adsorbed [38] , one can expose the NaCl surface to higher water pressure and perform the similar temperature-dependent experiments for future studies. Fölsch et al. [20] reported a puckered hexagonal c(4 × 2) bilayer structure on NaCl(001) surface by low energy electron diffraction (LEED) analysis, which is different from what we observed in this work. Our DFT calculations show that the adsorption energy of the c(4 × 2) structure is very similar to that of the tetramer-based 2D ice structure, suggesting that both structures are thermodynamically favoured. We notice that the deposition temperature in the LEED experiments is about 135–155 K, much higher than that in our experiment (77 K). Therefore, the different ice structures may result from the growth kinetics. At low temperature, the water molecules prefer to locally form tetramers owing to the low mobility, whereas at higher temperature the water gains enough thermal energy to escape the constraint of the substrate and tend to follow the bulk-like arrangement to optimize the water–water interaction. In conclusion, a combination of STM techniques and DFT calculations is used to study the clustering and wetting of water on NaCl(001) surface. A novel bridging mechanism facilitates the interconnection of tetramer units, leading to a new type of 2D bilayer ice structure. The formation of the periodic Bjerrum defects with unusually high density is strongly against the Bernal–Fowler–Pauling ice rules and may have a crucial role in catalysing heterogeneous chemical reactions on water-coated salt surfaces, as well as in influencing various phenomena such as heterogeneous ice nucleation, salt dissolution and caking. This work not only sheds new light on the microscopic understanding of water–salt interaction, but also introduces a new way to build up an unconventional bilayer ice, which may be general on hydrophilic surfaces with tetragonal symmetry as long as interactions of water molecules with the substrates are comparable to interactions between water molecules. STM experiments The experiments were performed with an ultra-high vacuum cryogenic (5 K) STM (Createc, Germany) with the base pressure better than 5 × 10 −11 Torr. The Au(111) single crystal was repeatedly sputtered with Ar + and annealed at ~900 K, until a clean Au(111)–22 × √3 reconstructed surface was obtained. The NaCl (Sigma-Aldrich, 99.999%) was then evaporated thermally from a Knudsen cell at a temperature of 720 K onto the Au(111) surface held at room temperature. The ultrapure H 2 O (Sigma-Aldrich, deuterium-depleted) was further purified under vacuum by freeze-thaw cycles to remove remaining impurities. The H 2 O molecules were dosed in situ onto the sample surface kept at 77 K with a rate of 0.02 BL min −1 through a dosing tube, which pointed towards the sample from a distance of ~6 cm. The subsequent STM measurements were performed both at 77 and 5 K with electrochemically etched tungsten tips, which were cleaned by alternative annealing and sputtering before the experiments, and further by controlled field-emission and tip-crash procedures during the scanning. Bias voltage refers to the sample voltage with respect to the tip. All the STM topographic images were obtained in the constant current mode. The STM results obtained at 77 and 5 K were essentially the same. Image processing was performed by Nanotec WSxM [39] . Ab initio calculations DFT calculations were performed using Vienna Ab-initio Simulation Package code (VASP) [40] , [41] to determine the stable adsorption structures of water clusters on NaCl(001) surface. Projector-augmented wave pseudopotentials [42] were used together with a plane wave basis set and a cutoff energy of 550 eV for the expansion of the electronic wave functions. Van der Waals corrections for dispersion forces were considered within the vdW-DF scheme by using the optB88-vdW method [43] , [44] . A bilayer NaCl(001) slab separated by a vacuum of 15-Å thick was used in the DFT simulation as the substrate for water adsorption. The bottom layer of the NaCl was fixed during the relaxation with the lattice constant of 5.665 Å. A Monkhorst–Pack grid with at least 8 × 8 × 1 k -point sampling per 1 × 1 cell was used. In the calculation of adsorption of water clusters, water/NaCl(001) structures were built with large unit cells to keep the error of water–image interaction at a negligible level. Adsorption energy was calculated by subtracting the total energy of the nH 2 O/NaCl(001) structure from the sum of the energies of the relaxed bare NaCl(001) substrate and n isolated water molecules in gas phase: Water–water interaction was estimated by the energy difference between the adsorbed water cluster in the absence of the NaCl substrate and n water molecules in gas phase: The water–substrate interaction was taken as the adsorption energy minus the water–water interaction: The adsorption of 2D ice was calculated using a 3 × 3 periodic tetramer-based bilayer ice slab on a 6 × 6 NaCl(001) substrate. Dozens of initial structures were generated with random distribution of tetramer chirality and Bjerrum-defect orientations. After performing structural relaxation, the order parameters were calculated afterwards as well as the total energies. Different models and methods were carefully tested to further support the validity of our DFT calculations (for details, see Supplementary Note 4 , Supplementary Fig. 4 and Supplementary Table 1 ). How to cite this article: Chen, J. et al. An unconventional bilayer ice structure on a NaCl(001) film. Nat. Commun. 5:4056 doi: 10.1038/ncomms5056 (2014).